Quantitative high throughput screening using a primary human three-dimensional organotypic culture predictsin vivoefficacy The tumour microenvironment contributes to cancer metastasis and drug resistance. However, most high throughput screening (HTS) assays for drug discovery use cancer cells grown in monolayers. Here we show that a multilayered culture containing primary human fibroblasts, mesothelial cells and extracellular matrix can be adapted into a reliable 384- and 1,536-multi-well HTS assay that reproduces the human ovarian cancer (OvCa) metastatic microenvironment. We validate the identified inhibitors in secondary in vitro and in vivo biological assays using three OvCa cell lines: HeyA8, SKOV3ip1 and Tyk-nu. The active compounds directly inhibit at least two of the three OvCa functions: adhesion, invasion and growth. In vivo , these compounds prevent OvCa adhesion, invasion and metastasis, and improve survival in mouse models. Collectively, these data indicate that a complex three-dimensional culture of the tumour microenvironment can be adapted for quantitative HTS and may improve the disease relevance of assays used for drug screening. The tumour microenvironment plays an important role in the processes of metastasis and drug resistance [1] , [2] , [3] , [4] , yet most drug discovery programmes involving high throughput screening (HTS) use cancer cells cultured in a monolayer two-dimensional (2D) on plastic [5] , [6] , [7] . The absence of surrounding stromal cells and extracellular matrix (ECM) in screening assays may provide one explanation for the high attrition rate of drugs as they transition into clinical testing. While assays using cells cultured on plastic can be useful for discovering small molecule inhibitors of proteins that promote carcinogenesis, they cannot reproduce the cellular heterogeneity, the complex architecture and the key interactions that occur within the tumour microenvironment in vivo . Single cell-type tumour spheroids are utilized infrequently in HTS. Though the spheroids can recapitulate some aspects of cancer cell growth in 3D, their variable growth patterns make them unsuitable for HTS [8] , [9] . Spheroids also cannot replicate bidirectional interactions between tumour cells, stromal cells and the ECM [10] , [11] , [12] , [13] . Interestingly, tumour cells grown in a multi-cell-type 3D organotypic model show significant differences in drug sensitivity when compared with cancer cells grown in single cell-type 3D spheroids or as a monolayer [11] . Treatment with a PI3-kinase or MAP kinase inhibitor blocked the proliferation of tumour cells grown in 2D. However, the same cells cultured in 3D showed a 10–100-fold reduction in sensitivity to the inhibitor, implying that the cellular context and a 3D environment has an important effect in drug resistance [14] , [15] . These results underscore the importance of performing screens for new drugs using model systems that more faithfully recapitulate tissue architecture at the metastatic site. Ovarian cancer (OvCa) is a very aggressive tumour of the female genital tract. No new drugs have been approved for OvCa treatment since 1999, when liposomal doxorubicin entered clinical care for recurrent disease [16] . One reason many chemotherapy drugs that successfully treat other epithelial cancers (for example, breast, colon) have not been effective in patients with OvCa might be the unusual metastatic pattern observed in advanced OvCa, which rarely metastasizes hematogenously [17] . Instead, tumour cells detach from the ovary and/or fallopian tube and are transported by the peritoneal fluid to the surfaces of organs in the abdominal cavity, where they establish metastatic colonies [18] , [19] . The principal sites of OvCa metastasis are the omentum, a large fat pad (~20 × 20 × 3 cm) that covers the bowel in the peritoneal cavity, and the peritoneum, the serous membrane that lines the peritoneal cavity [17] . In this study, our goal was to recapitulate the structural organization and function of the superficial tissue layers encountered by OvCa cells during metastasis in an assay amenable to drug screening using a HTS platform. Our hypothesis was that by adapting a 3D system that more faithfully represents the histologic and biologic complexity of the most common sites of OvCa metastasis for HTS, we could more reliably identify those compounds that effectively inhibit metastasis in vivo . We developed a heterotypic organotypic culture assay that mimics the surface histology of the omentum and peritoneum using primary cells, and used it to evaluate the effects of small molecule compounds on the adhesion, migration and invasion of OvCa cells. Our results demonstrate that an in vitro 3D model based on primary cells can be used effectively in HTS and could become an important tool for improving drug screening efficacy. Establishment of an organotypic HTS assay All organs in the peritoneal cavity are covered by a single layer of mesothelial cells that rest on a basement membrane of ECM interspersed with fibroblasts ( Fig. 1a ) [20] . A heterotypic, 3D organotypic culture assay mimicking the surface histology of the omentum and peritoneum was assembled with primary human mesothelial cells and fibroblasts mixed with ECM (fibronectin and collagen type I). The fibroblasts and mesothelial cells were isolated from human omental tissue obtained from women undergoing surgery for non-malignant conditions [21] . In culture, the fibroblasts and mesothelial cells maintained vimentin and cytokeratin expression patterns, respectively, ( Supplementary Fig. 1a ) as observed in vivo [21] . Fluorescent images exemplify the 3D localization of the OvCa cells (right panel, green) on top of the organotypic model containing mesothelial cells (blue) and fibroblasts (red) ( Fig. 1b ). The unlabelled 3D culture was then used to evaluate the effects of pharmacologically active compounds on the adhesion and invasion of two fluorescently labelled OvCa cells ( Fig. 1c ; Supplementary Fig. 1b ). 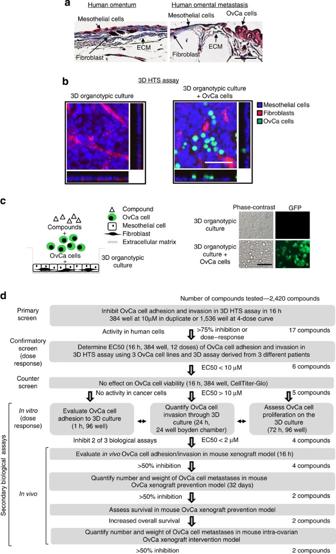Figure 1: Optimization of a 3D organotypic HTS assay designed to identify inhibitors of ovarian cancer adhesion and invasion. (a) Haematoxylin and eosin stained images of human omentum (left panel) and omental metastases (right panel; size bar, 50 μm). (b) Fluorescent images of the 3D HTS assay with fluorescently labelled mesothelial cells (blue, CMAC) and fibroblasts (red, CMPTX) with (right panel) and without SKOV3ip1 OvCa cells (green, CMFDA; left panel). Size bar, 100 μm.z-axis (45 μm) reconstruction of optical sections with orthogonal view of maximum intensity shown. (c) Schematic, phase and fluorescent images of the 3D organotypic HTS assay with and without fluorescently labelled (GFP) SKOV3ip1 OvCa cells in a 384-well plate (size bar, 100 μm). (d) Flow chart for 3D HTS screening platform including the primary, confirmatory, counter and secondary biological assays (in vitroandin vivo). The criteria for compound selection and the number of compounds at each step are listed. Figure 1: Optimization of a 3D organotypic HTS assay designed to identify inhibitors of ovarian cancer adhesion and invasion. ( a ) Haematoxylin and eosin stained images of human omentum (left panel) and omental metastases (right panel; size bar, 50 μm). ( b ) Fluorescent images of the 3D HTS assay with fluorescently labelled mesothelial cells (blue, CMAC) and fibroblasts (red, CMPTX) with (right panel) and without SKOV3ip1 OvCa cells (green, CMFDA; left panel). Size bar, 100 μm. z -axis (45 μm) reconstruction of optical sections with orthogonal view of maximum intensity shown. ( c ) Schematic, phase and fluorescent images of the 3D organotypic HTS assay with and without fluorescently labelled (GFP) SKOV3ip1 OvCa cells in a 384-well plate (size bar, 100 μm). ( d ) Flow chart for 3D HTS screening platform including the primary, confirmatory, counter and secondary biological assays ( in vitro and in vivo ). The criteria for compound selection and the number of compounds at each step are listed. Full size image The HTS assay was adapted into a 384-well format through optimization of several parameters, including the incubation time (16 h), number of cancer cells (12,000), mesothelial cells (4,000) and fibroblasts (400) ( Supplementary Fig. 2a–c ). Given that most small molecule compounds for drug screening are dissolved in dimethyl sulfoxide (DMSO), we tested the ability of the 3D culture to tolerate a range of concentrations of this solvent. Our results indicated that the 3D culture readily tolerated up to 1% DMSO ( Supplementary Fig. 2d ). The performance of the HTS assay was very reproducible on different days and with primary cells from different patients ( Supplementary Fig. 3a,b ). Most importantly, known inhibitors of OvCa adhesion and invasion (for example, integrin antibodies and arginine–glycine–aspartic acid peptides) blocked adhesion/invasion in the 3D culture ( Supplementary Fig. 3c ). As expected, platinum and taxanes, the OvCa chemotherapies that are used clinically to block proliferation [22] , did not inhibit OvCa cell adhesion and invasion in the 3D culture (half-maximal effective concentration (EC 50 ) of carboplatin, 176–255 μM; cisplatin, 52–58 μM; docetaxel, 30–43 μM and paclitaxel, 23–36 μM; Supplementary Fig. 3d ). These results suggest that by evaluating behaviours other than cell proliferation, we could identify inhibitors of OvCa metastasis that may not be revealed using traditional screening approaches. Careful optimization of the protocol enabled us to establish an 8-step, fully automated, 3D HTS assay in both 384- and 1,536-well formats ( Fig. 2a,b , Supplementary Figs 4,5 ). The 1,536-well format is advantageous because it requires 90% less volume and fewer primary cells than the 384-well format, allowing the screening of a larger collection of compounds. The 1,536-well format also permits a quantitative HTS approach that uses an automated, robotic system to screen the large collection of compounds in a 4-point dose response [23] . This reduces the number of false positive hits and enables the identification of compounds that are less potent, but are still potentially relevant [24] . 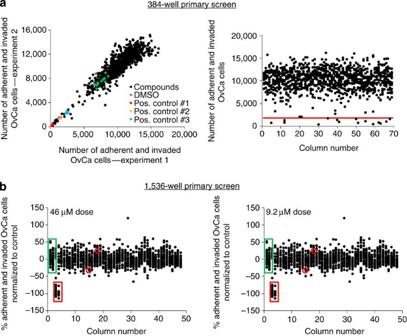Figure 2: The primary 3D organotypic HTS in 384-well and 1,536-well formats. (a) HTS assay (384 well). The Prestwick Chemical Library of compounds at a final concentration of 10 μM (n=2 experiments, 1,140 compounds) was added to the 384-well 3D HTS assay. Adhesion and invasion of SKOV3ip1–GFP cells after 16 h was evaluated using a fluorescence cytometer. Left, reproducibility plot of primary screen. Right, active compounds were defined as >75% inhibition of OvCa adhesion and invasion (below red line, 15 compounds total, 1% hit rate). (b) 1,536-well HTS assay (four dose responses; 46, 9.2, 1.8 and 0.36 μM). Adhesion and invasion of SKOV3ip1–GFP cells after 16 h was evaluated using a fluorescence cytometer. The 46- and 9.2-μM compound concentraion assay plates are shown. Active compounds were selected using a combination of parameters including curve response, class scoring, maximum response, efficacy and EC50 values (red circles, two compounds total, and 0.2% hit rate). The controls, DMSO (green box) and tomatine (red box) are shown. Pos., positive. Figure 2: The primary 3D organotypic HTS in 384-well and 1,536-well formats. ( a ) HTS assay (384 well). The Prestwick Chemical Library of compounds at a final concentration of 10 μM ( n =2 experiments, 1,140 compounds) was added to the 384-well 3D HTS assay. Adhesion and invasion of SKOV3ip1–GFP cells after 16 h was evaluated using a fluorescence cytometer. Left, reproducibility plot of primary screen. Right, active compounds were defined as >75% inhibition of OvCa adhesion and invasion (below red line, 15 compounds total, 1% hit rate). ( b ) 1,536-well HTS assay (four dose responses; 46, 9.2, 1.8 and 0.36 μM). Adhesion and invasion of SKOV3ip1–GFP cells after 16 h was evaluated using a fluorescence cytometer. The 46- and 9.2-μM compound concentraion assay plates are shown. Active compounds were selected using a combination of parameters including curve response, class scoring, maximum response, efficacy and EC50 values (red circles, two compounds total, and 0.2% hit rate). The controls, DMSO (green box) and tomatine (red box) are shown. Pos., positive. Full size image Our data shows that miniaturization of the organotypic assay from 384- to 1,536-well formats did not compromise the quality of the HTS assay. Both formats were highly robust and reproducible with signal-to-background ratios of 2.1–4.4 and Z -factors of 0.4–0.7 ( Supplementary Fig. 6a,b ), which are desirable for HTS [25] . We also found that the 384- and 1,536-well assay formats produce comparable results. Four active compounds, originally identified in the 384-well primary screen of the Prestwick Chemical Library (Prestwick), were tested in the 1,536-well format in an 11-point dose response. The dose–response curves showed that the EC50 values are comparable in the two formats ( Fig. 3 and Supplementary Fig. 6c ). Furthermore, the Library of Pharmacologically Active Compounds (LOPAC 1280 ) was screened at 46 μM in the 384-well format, and the per cent activity value of compounds was directly compared with the maximum dose, 46 μM, of the 1,536-well primary screen. A positive correlation between the experimental compounds was observed, and the controls, DMSO and tomatine clustered at 0% and −100% activity values, respectively ( Supplementary Fig. 6d ). 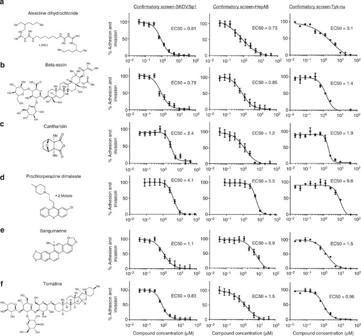Figure 3: Dose-dependent confirmation of active compounds. Adhesion and invasion of fluorescently labelled (GFP) SKOV3ip1, HeyA8 and Tyk-nu OvCa cells in the 3D culture (HTS assay) was measured over 16 h in a 384-well assay using a 12 dose curve for (a) alexidine dihydrochloride, (b) beta-escin, (c) cantharidin, (d) prochlorperazine dimaleate, (e) sanguinarine and (f) tomatine. Each curve represents the percentage of OvCa–GFP cells that invaded and adhered to the 3D culture. Data points represent mean±s.e.m. Figure 3: Dose-dependent confirmation of active compounds. Adhesion and invasion of fluorescently labelled (GFP) SKOV3ip1, HeyA8 and Tyk-nu OvCa cells in the 3D culture (HTS assay) was measured over 16 h in a 384-well assay using a 12 dose curve for ( a ) alexidine dihydrochloride, ( b ) beta-escin, ( c ) cantharidin, ( d ) prochlorperazine dimaleate, ( e ) sanguinarine and ( f ) tomatine. Each curve represents the percentage of OvCa–GFP cells that invaded and adhered to the 3D culture. Data points represent mean±s.e.m. Full size image A methodical screening approach was employed to evaluate the effect of small molecule compounds on the early steps of OvCa metastasis ( Fig. 1d ). Inhibition of fluorescently labelled OvCa cell adhesion/invasion to the organotypic HTS assay was evaluated in a primary screen, followed by confirmation of ‘hit’ compounds in expanded dose–response curves. A counter screen was used to eliminate compounds that were toxic to cells during the 3D HTS assay. Three independent secondary in vitro biological assays validated the effect of each compound on OvCa cell adhesion, invasion and growth. Finally, four different in vivo functional assays were performed, adhesion/invasion, metastasis prevention, survival prevention and intra-ovarian metastasis intervention assays, to identify compounds with in vivo efficacy. Implementation of a 3D organotypic quantitative HTS platform The Prestwick and the LOPAC 1280 were screened using the 3D HTS culture model to identify compounds that inhibit the key steps of early metastasis. These two libraries of compounds are the most widely used assay validation libraries. They contain all major drug target classes and high chemical and pharmacological diversity [26] . The 1,140 compounds of the Prestwick library were screened in a 384-well format at a concentration of 10 μM ( Fig. 2a ). The reproducibility plot of this 384-well format screen (left panel) and a scatter plot of the number of adherent and invaded OvCa cells in each column (right panel) illustrate the quality of this assay. The 1,280 compounds of the LOPAC 1280 library were screened in a 1,536-well format at 4 doses—46, 9.2, 1.8 and 0.36 μM. Examples of the quantitative HTS assay performance is shown in Fig. 2b as scatter plots from the top two doses of compounds tested (46 and 9.2 μM) after data normalization according to DMSO basal (0% inhibition, columns 1 and 2) and tomatine control (−100% inhibition, columns 3 and 4, rows 1–16). The signal-to-background ratio was 4.1 and 3.7, the Z′-factor was 0.58 and 0.62 for 46 μM and 9.2 μM plates, respectively, indicating that the assay was robust for 1,536-well quantitative HTS. Using the Prestwick library in the 384-well format, we identified 15 compounds that inhibited adhesion and invasion of OvCa cells by at least 75% (3s.d. calculated relative to the control wells treated with DMSO; below the red line in the right panel, Fig. 2a ). We identified 2 additional compounds using the LOPAC 1280 library screen in 1,536-well format. These compounds were reconfirmed in the 3D HTS assay using an 11-point response. The dose-dependent inhibition curves are shown in Supplementary Fig. 7 . The 17 identified compounds were tested in multi-dose 384-well confirmatory screens ( Fig. 3a–f , Supplementary Figs 8,9 ). In these screens, compounds with no response or with an EC 50 >10 μM were considered inactive ( Supplementary Figs 8,9 ), while compounds with EC 50 values ≤10 μM were considered active ( Fig. 3a–f ), and were, therefore, further evaluated. Six out of the initial 17 compounds identified using the Prestwick and LOPAC compound libraries were active in three OvCa cell lines, SKOV3ip1, HeyA8 and Tyk-nu, in the 3D culture assay. A counter screen was performed to identify and eliminate compounds that affected OvCa cell viability within the time of the assay ( Supplementary Fig. 10 ). SKOV3ip1, HeyA8 or Tyk-nu cells were cultured on plastic and treated with the compounds at concentrations of 1, 5 or 10 μM, and cell viability was measured after 16 h. Five of the 6 compounds (alexidine dihydrochloride, beta-escin, cantharidin, prochlorperazine dimaleate and tomatine) had no effect on viability at 16 h (EC 50 >10 μM). Next, the effect of these five compounds on cell viability after 72 h of treatment was evaluated with the intention of prioritizing compounds that also inhibit OvCa viability after long-term treatment ( Supplementary Fig. 11 ). SKOV3ip1, HeyA8 or Tyk-nu cells were cultured on plastic and treated with the compounds at concentrations of 1, 5 or 10 μM, and cell viability was measured after 72 h. All five compounds (alexidine dihydrochloride, beta-escin, cantharidin and tomatine) inhibited OvCa cell viability after 72 h of treatment on plastic. The five compounds were then tested in three functional screens using SKOV3ip1, HeyA8 and Tyk-nu OvCa cell lines at three different doses ( Fig. 4a–c ). Four compounds (alexidine dihydrochloride, beta-escin, cantharidin and tomatine) inhibited adhesion to the 3D organotypic culture after 1 h ( Fig. 4a ). Three compounds (beta-escin, cantharidin and tomatine) inhibited OvCa cell invasion through the 3D organotypic culture after 24 h ( Fig. 4b ). Finally, two compounds (cantharidin and prochlorperazine dimaleate) decreased OvCa cell growth after 72 h when co-cultured with the 3D organotypic culture ( Fig. 4c ). Because four compounds (alexidine dihydrochloride, beta-escin, cantharidin and tomatine) significantly inhibited at least two key OvCa functions in early metastasis at a low dose (1 μM), we evaluated the efficacy of these compounds in vivo . 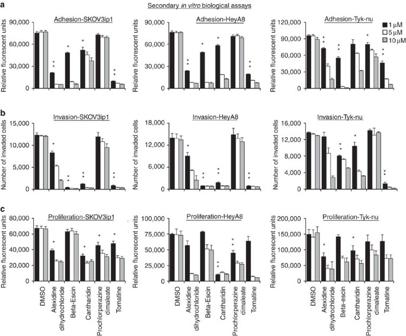Figure 4:In vitrovalidation of active compounds. Secondaryin vitrobiological assays using fluorescently labelled (GFP) SKOV3ip1, HeyA8 and Tyk-nu OvCa cells. Each compound was tested at 1, 5 and 10 μM concentrations or an equal volume of DMSO at each dose. (a) Adhesion assay. The adhesion of OvCa–GFP cells to the 3D culture (n=5, 96 well) was measured using a fluorescent plate reader. (b) Invasion assay. The invasion of OvCa–GFP cells through the 3D culture plated on a 24-well transwell (n=5) was analyzed by fluorescent microscopy. (c) Cell growth assay. The growth of OvCa–GFP cells on the 3D culture after 72 h (n=5, 96 well) was detected using a fluorescent plate reader. Bars represent mean±s.e.m. Significant changes were determined by two-sided unpairedt-tests. *P<0.05, **P<0.001. Figure 4: In vitro validation of active compounds. Secondary in vitro biological assays using fluorescently labelled (GFP) SKOV3ip1, HeyA8 and Tyk-nu OvCa cells. Each compound was tested at 1, 5 and 10 μM concentrations or an equal volume of DMSO at each dose. ( a ) Adhesion assay. The adhesion of OvCa–GFP cells to the 3D culture ( n =5, 96 well) was measured using a fluorescent plate reader. ( b ) Invasion assay. The invasion of OvCa–GFP cells through the 3D culture plated on a 24-well transwell ( n =5) was analyzed by fluorescent microscopy. ( c ) Cell growth assay. The growth of OvCa–GFP cells on the 3D culture after 72 h ( n =5, 96 well) was detected using a fluorescent plate reader. Bars represent mean±s.e.m. Significant changes were determined by two-sided unpaired t -tests. * P <0.05, ** P <0.001. Full size image Validation of active hits and analysis of in vivo efficacy To validate the in vitro results, we evaluated the effect of early treatment (prevention study) with each compound in three in vivo assays. First, we performed a short-term adhesion/invasion assay in the mouse peritoneal cavity [27] , [28] , using the same 16 h time point used in the in vitro studies. Fluorescently labelled SKOV3ip1 or HeyA8 OvCa cells were mixed with each of the four lead compounds (alexidine dihydrochloride, beta-escin, cantharidin and tomatine), injected intra-peritoneally (i.p.) into mice and cancer cell adhesion/invasion was measured. Consistent with the in vitro studies, all four compounds inhibited adhesion/invasion to the peritoneal surface and omentum in vivo ( Fig. 5a , Supplementary Fig. 12 ). We next performed a metastasis assay using a SKOV3ip1 xenograft mouse model [20] , [27] , [29] , [30] . The mice were injected i.p. with SKOV3ip1 cells mixed with each of the four compounds, and the treatment was continued on days 2 and 4. The early i.p. treatment of mice with beta-escin and tomatine, prior to OvCa cell implantation on the intra-abdominal surface, resulted in inhibition of tumour growth and metastasis by 96% when compared with control mice. Alexidine dihydrochloride and cantharidine were less effective than beta-escin and tomatine, but still reduced tumour growth and metastasis by >35% ( Fig. 5b ). Third, we performed survival assays [20] in which mice were i.p. injected with either SKOV3ip1 or HeyA8 OvCa cells using the same treatment schedule as shown in Fig. 5b . In both xenograft models the treatment of mice with beta-escin and tomatine ( Fig. 5c ) increased overall survival significantly (100% alive on day 65 in both models) compared with vehicle-treated control mice (median survival for SKOV3ip1: 29.5 days; median survival for HeyA8: 20 days). 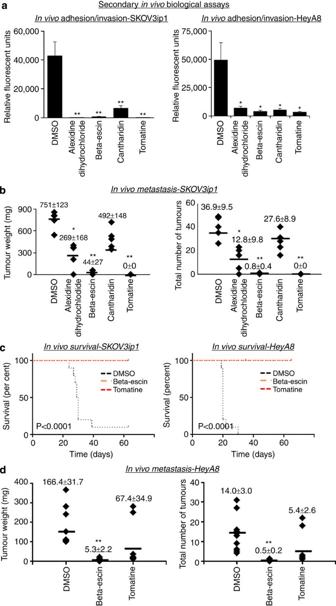Figure 5:In vivovalidation of active compounds. Secondaryin vivobiological assays using fluorescently labelled (GFP) SKOV3ip1 and HeyA8 OvCa cells. (a)In vivoadhesion and invasion assay. Four million OvCa–GFP cells were injected i.p., and 16 h later the omentum was collected. Bound OvCa cells were digested from the omentum and total fluorescence was quantified using a fluorescent plate reader (n=5). (b)In vivoprevention study. One million SKOV3ip1 cells were injected i.p. with compounds or DMSO (5 μM), and i.p. treatment continued at 48 and 96 h post-cancer cell injection (10 mg kg−1,n=5). Tumours were collected 32 days post-cancer cell injection and weighed. Significant changes were determined by two-sided unpairedt-tests. *P<0.05, **P<0.001. (c)In vivosurvival study. One million OvCa cells were injected i.p. with beta-escin, tomatine or DMSO (5 μM), and i.p. treatment continued at 48 and 96 h post-cancer cell injection (10 mg kg−1or equal volume of DMSO,n=5). Mice were killed once they showed signs of distress, and Kaplan–Meier curves were calculated. (d)In vivointra-ovarian intervention study. Twenty-five thousand OvCa cells were injected intra-ovarian; 7 days post-injection treatment started with beta-escin, tomatine (1 mg kg−1,n=10) or DMSO (volume control) and i.p. treatment continued three times a week for 2 weeks. Figure 5: In vivo validation of active compounds. Secondary in vivo biological assays using fluorescently labelled (GFP) SKOV3ip1 and HeyA8 OvCa cells. ( a ) In vivo adhesion and invasion assay. Four million OvCa–GFP cells were injected i.p., and 16 h later the omentum was collected. Bound OvCa cells were digested from the omentum and total fluorescence was quantified using a fluorescent plate reader ( n =5). ( b ) In vivo prevention study. One million SKOV3ip1 cells were injected i.p. with compounds or DMSO (5 μM), and i.p. treatment continued at 48 and 96 h post-cancer cell injection (10 mg kg −1 , n =5). Tumours were collected 32 days post-cancer cell injection and weighed. Significant changes were determined by two-sided unpaired t -tests. * P <0.05, ** P <0.001. ( c ) In vivo survival study. One million OvCa cells were injected i.p. with beta-escin, tomatine or DMSO (5 μM), and i.p. treatment continued at 48 and 96 h post-cancer cell injection (10 mg kg −1 or equal volume of DMSO, n =5). Mice were killed once they showed signs of distress, and Kaplan–Meier curves were calculated. ( d ) In vivo intra-ovarian intervention study. Twenty-five thousand OvCa cells were injected intra-ovarian; 7 days post-injection treatment started with beta-escin, tomatine (1 mg kg −1 , n =10) or DMSO (volume control) and i.p. treatment continued three times a week for 2 weeks. Full size image Finally, we evaluated the effect of the two most promising compounds, beta-escin and tomatine, on OvCa metastasis after tumour establishment (intervention study) [27] . In this experiment, mice received intra-ovarian injections of HeyA8 OvCa cells, and after the metastatic disease was established (7 days) mice received six i.p. treatments (3 days per week) with beta-escin or tomatine ( Fig. 5d ). Treatment with beta-escin resulted in inhibition of tumour growth and metastasis by 97% when compared with control mice. Tomatine was less effective than beta-escin, but still reduced tumour growth and metastasis by >59%. In summary, our data demonstrate the ability of the 3D HTS assay to predict the efficacy of small molecule compounds in vivo . Specifically, the compounds that showed the highest activity in in vitro studies were similarly effective in preventing metastasis in in vivo mouse studies. We have developed a human organotypic assay that recreates key features of the OvCa tumour microenvironment encountered by cells metastasizing to the peritoneum and omentum. This new platform allows us to perform consistent, reproducible and quantitative HTS campaigns in a context that mimics the biology of OvCa. Orthotopic primary human stromal cells were mixed with ECM proteins to re-construct, in vitro , the superficial tissue layers of the omental and peritoneal surfaces, which are the principal sites of OvCa metastasis in vivo [17] , [18] , [19] . In screens using this assay in 384- and 1,536-well formats, we successfully identified small molecule inhibitors of the early steps of OvCa metastasis. The compounds, which blocked adhesion, migration, invasion and/or growth in the 3D model and inhibited OvCa cell viability at 72 h, were confirmed in four unique in vivo assays with two different cell lines. These results showed that the 3D HTS platform has a high predictive value for in vivo efficacy. One small molecule compound identified in the screens, beta-escin, very efficiently inhibited the adhesion, migration, invasion and viability of OvCa cells in vitro. This in vitro activity was mirrored by an inhibition of in vivo adhesion, which translated into the formation of fewer metastatic nodules. Indeed, tumour load was very efficiently reduced (>94%) in mice treated with beta-escin when compared with control mice in the prevention and intervention treatment studies. Beta-escin (Venastat) is a natural mixture of triterpenoid saponins (horse chestnut) that has previously been shown to improve chronic venous insufficiency. In addition, it sensitizes cells in culture to gemcitabine chemotherapy and inhibits NF-κB signalling [31] . It is conceivable that beta-escin, which is highly effective in preventing early OvCa metastasis, may also be useful for the treatment of other cancers that metastasize to the same anatomic sites within the peritoneal cavity, such as gastric, colon and pancreatic cancer. Our goal was to recapitulate the OvCa metastatic microenvironment in vitro to investigate OvCa cell adhesion/invasion. While the 3D HTS platform does not fully reproduce this in vivo environment, it has several important advantages. First, it has a modular design that facilitates incorporation of any cell type present in the tumour microenvironment. In the OvCa metastatic environment, these cells include adipocytes, various immune cells and endothelial cells [28] . Second, primary human cancer cells or tumour cell spheroids isolated from ascites or solid tumours can be integrated into the platform [32] . In addition, ascites fluid, which provides a pro-inflammatory and tumour-promoting environment and is present in over a third of all OvCa patients when diagnosed, can be incorporated into the 3D culture to screen for therapeutic agents that target ascites-driven effects. Moreover, the culture can be customized to screen for therapeutic agents that target specific metastatic sites, including secondary sites, by using primary stromal cells common to that particular microenvironment. For example, the metastatic microenvironment of breast cancer in the lung, bone or liver could be investigated by incorporating activated bone marrow-derived cells, endothelial cells, pericytes and other organ-specific cells [33] . Cell-based assays can be difficult to scale for HTS, and the use of primary human cells in HTS has been limited because the cells are challenging to culture [7] , [9] . However, we found that primary human cells can be successfully cultured, adapted and scaled to dependable and consistent 384-well and 1,536-well formats. In fact, our screens had high Z′-factors, comparable to those of ‘simpler’ screening approaches that use one cell line on plastic. Sophisticated 3D models, designed to recapitulate the natural tumour composition, can bridge the gap between 2D cell proliferation assays and animal models [34] . Indeed, they may reduce the need for animal testing, since they provide a biologically relevant platform for screening compounds. Moreover, these models are particularly suited to personalized medicine because primary patient-derived cells can be used when testing thousands of compounds in real time. In summary, our results suggest that drug discovery using physiologically applicable organotypic models for human disease is practical, and likely to identify effective drugs more quickly and with a lower attrition rate than other screening approaches. Reagents The LOPAC 1280 was obtained from Sigma-Aldrich (1,280 pharmacologically active small molecules including marketed drugs and pharmaceutically relevant structures annotated with biological activities). The Prestwick Chemical Library (1,140 small molecule drugs, 100% approved by Food and Drug Administration (FDA), European Medicines Agency (EMEA) and other agencies) was purchased from Prestwick Chemical. The active compounds were re-purchased from independent sources. Alexidine dihydrochloride (CAS 171530-6), beta-escin (CAS 6805-41-0) and cantharidin (CAS 56-25-7) were from Sigma-Aldrich, and sanguinarine (CAS 5578-73-4), prochlorperazine dimaleate (CAS 84-02-6) and tomatine (CAS 17406-45-0) were from Tocris Bioscience. CellTracker Green (CMFDA), Red (CMPTX) and blue (CMAC) were purchased from Life Technologies. The MMP inhibitor, GM6001 (EMD Bioscience), vimentin antibody (1:600 dilution, clone M0725, Dako Cytomation), cytokeratin 8 antibody (1:500 dilution, clone Ks8.7, Santa Cruz Biotechnology), collagen type I and fibronectin were purchased from BD Biosciences. The Arg–Gly–Asp and Arg–Ala–Asp peptides were from Sigma-Aldrich. Cell lines The human OvCa cell lines, SKOV3ip1 and HeyA8, were provided by Dr Gordon B. Mills (MD Anderson Cancer Center), and are cultured in DMEM with 10% foetal bovine serum, 1% penicillin–streptomycin and 1% L -glutamine. The Tyk-nu cells were provided by Dr Kenjiro Sawada (Osaka University), and are cultured in EMEM with 15% foetal bovine serum, 1% penicillin–streptomycin and 1% L-glutamine. The cells were validated by short tandem repeat DNA fingerprinting using the AmpFℓSTR Identifier kit (Applied Biosystems) and compared with known American Type Culture Collection fingerprints, the Cell Line Integrated Molecular Authentication database (CLIMA) and the University of Texas MD Anderson Cancer Center fingerprint database. The green fluorescent protein (GFP)-labelled OvCa cells were constructed utilizing a lentivirus vector expressing copepod GFP (CD511B-1) and the lentivirus packing kit (LV500A-1) [35] . The lentivirus vector expressing copepod (c)GFP (CD511B-1) and the lentivirus packaging kit (LV500A-1) were purchased from System Biosciences (Mountain View, CA, USA). Primary 3D HTS Specimens of fresh human omentum were obtained from patients undergoing surgery for benign conditions and those who provided informed consent before surgery. The protocol was approved by the University of Chicago Biological Sciences Division/the University of Chicago Medical Center Institutional Review Board. Primary human mesothelial cells and fibroblasts were isolated from normal human omentum and purity was verified by vimentin and cytokeratin immunohistochemistry ( Supplementary Fig. 1a ) [20] , [21] . All primary human fibroblasts and mesothelial cells were used within the first two passages after isolation. All primary human cells were collected and stored in liquid nitrogen immediately after isolation for utilization in screens. For the 384-well format, primary human omental fibroblasts (400) and mesothelial cells (4,000) were seeded with 0.2 μg fibronectin and 0.2 μg collagen type I in 40 μl of growth media (0.06 cm 2 , Supplementary Fig. 4 ). After 48 h of incubation at 37 °C/5% CO 2 /95% relative humidity, SKOV3ip1–GFP OvCa cells (12,000) were seeded in 40 μl of serum-free media (growth media minus foetal bovine serum) on top of primary human omental cells. In the Prestwick library screen, the library compounds dissolved in DMSO at 10 μM final concentration, positive controls (arginine–glycine–aspartic acid peptide, MMP inhibitor or tomatine) at 10 μM final concentration or DMSO (0.4 μl, equal volume control) were added to each well immediately after the addition of cancer cells. In the LOPAC 1280 screen, the library compounds dissolved in DMSO at 46 μM final concentration, positive control (tomatine) at 10 μM final concentration or DMSO (0.4 μl, equal volume control) were added to each well immediately after the addition of cancer cells. The plates were incubated at room temperature for 2 h before being placed in an incubator at 37 °C. After 16 h of incubation, each well was washed with phosphate-buffered saline (PBS, 40 μl). PBS was aspirated and each well was fixed with 4% paraformaldehyde (PFA). The number of fluorescent cells in the assay was analyzed using a fluorescent cytometer (TTP Labtech Acumen eX3). For the 1,536-well format, 40 primary human omental fibroblasts and 400 mesothelial cells were seeded with 0.02 μg fibronectin and 0.02 μg collagen type I in 4 μl of growth media (2.3 mm 2 , Supplementary Fig. 5 ). After 48 h of incubation at 37 °C, 1,200 SKOV3ip1–GFP or HeyA8–GFP OvCa cells were seeded in 3 μl of serum-free media (growth media minus foetal bovine serum) on top of primary human omental cells. The (LOPAC 1280 ) library of compounds was screened in four doses (0.36–46 μM), and the plates contained the positive control (tomatine) in eight doses (0.035–75 μM) and DMSO (equal volume controls). The compounds or controls were added to each well immediately after addition of the cancer cells. The plates were incubated at room temperature for 2 h and then at 37 °C for 16 h. Following incubation, the media was aspirated and each well was washed with PBS (5 μl) and then fixed with 4% PFA (5 μl). After 20 min, the PFA solution was aspirated, PBS (5 μl) was added and the number of fluorescent cells was analyzed using a fluorescent cytometer. Confirmatory, counter and 72-h viability assays. The 3D HTS assay was plated in a 384-well format, and after 48 h of incubation 12,000 OvCa cells were seeded in 40 μl of serum-free media on top of primary human omental mesothelial cells (4,000) and fibroblasts (400). The dose response of the compounds was tested (40–40 μM). The compounds dissolved in DMSO or DMSO (equal volume control) was added to each well immediately after the addition of cancer cells. The plates were incubated, treated and fixed as described above and the number of fluorescent cells was analyzed using a fluorescent cytometer. For the counter assay, OvCa cells, 4,000 SKOV3ip1 or 2,000 HeyA8, were seeded in 40 μl of growth media and incubated for 24 h. Compounds dissolved in DMSO at doses of 1, 5 or 10 μM or DMSO (equal volume control) were added. The plates were incubated at room temperature for 2 h before being placed in an incubator at 37 °C. After 16 h of incubation at 37 °C, the CellTiter-Glo cell viability assay (Promega) was performed and analyzed using a luminescent plate reader (Molecular Devices Analyst GT). For the 72 h viability assay, OvCa cells, 1,000 SKOV3ip1 or 500 HeyA8 were seeded in 40 μl of growth media and incubated for 24 h. Compounds dissolved in DMSO at doses of 1, 5 or 10 μM or DMSO (equal volume control) were added. The plates were incubated at room temperature for 2 h before being placed in an incubator at 37 °C. After 72 h of incubation at 37 °C, the CellTiter-Glo assay was performed. Secondary biological in vitro assays The 3D culture was assembled on black-walled 96-well plates for adhesion and growth assays. For invasion assays, the 3D culture was assembled on pre-coated (15 μg of collagen type I) 24-well transwell inserts (BD Biosciences) [20] , [21] . Compounds dissolved in DMSO were tested at 1, 2, 5 and 10 μM concentrations, and DMSO (equal volumes) was the control. For a 1 h adhesion assay, 40,000 fluorescently labelled SKOV3ip1–GFP, HeyA8–GFP or Tyk-nu–GFP OvCa cells were mixed with the compounds and seeded in 100 μl of serum-free media on top of the 3D culture (0.33 cm 2 , n =5). After 1 h of incubation at 37 °C, the wells were washed with PBS, fixed with PFA and cell fluorescence was detected using a fluorescent plate reader (Synergy HT). For the invasion assay, 50,000 SKOV3ip1–GFP, HeyA8–GFP or Tyk-nu–GFP cells were seeded in 100 μl of serum-free media in the upper chamber of a 24-well transwell plate (0.33 cm 2 , n =3) pre-coated with the 3D culture [20] . The compounds were added to the cancer cells in the upper chamber, growth media (700 μl) was placed in the bottom chamber and the plates were incubated at 37 °C for 24 h. All cells were removed from the top chamber and the invaded OvCa cells were quantified using a fluorescent microscope (× 10 objective, 5-fields for each transwell). For the cell growth assay, 4,000 SKOV3ip1–GFP, HeyA8–GFP or Tyk-nu–GFP cells were seeded in 100 μl of serum-free media on top of the 3D culture (0.33 cm 2 , n =5). The compounds were added after 30 min, the plates were incubated for 72 h at 37 °C, and the total fluorescence of cells was analyzed using a fluorescent plate reader. Animal experiments Female Harlan-Sprague Dawley: athymic Nude- Foxn1 nu mice of age 5–6 weeks and weighing ~20 g were purchased from Harlan Laboratories. All procedures involving animal care were approved by the Committee on Animal Care at the University of Chicago. In vivo adhesion/invasion assay Mice were injected i.p. with four million SKOV3ip1–GFP or HeyA8–GFP cells mixed with compounds (5 μM) or DMSO (equal volume). Sixteen hours (the same time span as the primary screen) after cancer cell injection, the mice were killed (five mice per group). The omentum was removed and imaged using fluorescent microscopy. The OvCa cells were digested off from the omentum by scraping and digesting in 1% nonyl phenoxypolyethoxylethanol in PBS for 1 h at 37 °C. The cells were collected, spun down and the total fluorescence (excitation: 488nm, emission: 520 nm) of the cells was analyzed using a fluorescent plate reader. In vivo prevention assay Mice were injected i.p. with SKOV3ip1 cells (1 × 10 6 ) mixed with compounds (5 μM) or DMSO (equal volume) on day 1 (five mice per group). Mice were treated twice after inoculation (48 and 96 h) with i.p. injection of compounds (1 mg kg −1 per day) in PBS (200 μl). Thirty-two days after injection, the mice were killed (five mice per group) [20] . The tumour colonies were counted, collected and weighed. In vivo prevention survival assay Mice were injected i.p. with SKOV3ip1 or HeyA8 cells (1 × 10 6 ) mixed with compounds (5 μM) or DMSO (equal volume) on day 1. Mice were treated twice after inoculation (48 and 96 h) with i.p. injection of compounds (1 mg kg −1 per day) in PBS (200 μl). The mice (10 per group) were killed at the first signs of distress [20] . Orthotopic intra-ovarian injection of tumour cells HeyA8 cells (2.5 × 10 5 ) were injected into the ovary of nude female mice. Seven days after inoculation (intervention study), mice were treated three times a week by i.p. injection of compounds (1 mg kg −1 per day) in PBS (200 μl). Twenty-one days after injection, the mice were killed (10 mice per group) [20] , [27] . The tumour colonies were counted, collected and weighed. Statistical analysis Confirmatory assay ( n =10), adhesion ( n =5), invasion ( n =3) and growth ( n =5) assays were performed and at least three independent experiments were conducted. The mean and s.e.m. are reported. Significant changes were determined by two-sided unpaired t -tests. Kaplan–Meier survival estimates were calculated to determine significant changes in the survival study. How to cite this article : Kenny, H. A. et al . Quantitative high throughput screening using a primary human three-dimensional organotypic culture predicts in vivo efficacy. Nat. Commun. 6:6220 doi: 10.1038/ncomms7220 (2015).